Herpesviruses carrying a Brainbow cassette reveal replication and expression of limited numbers of incoming genomes Whether all the infectious herpesvirus particles entering a cell are able to replicate and/or express their genomes is not known. Here, we developed a general method to determine the number of viral genomes expressed in an infected cell. We constructed and analysed fluorophore expression from a recombinant pseudorabies virus (PRV263) carrying a Brainbow cassette (Cre-conditional expression of different fluorophores). Using three isogenic strains derived from PRV263, each expressing a single fluorophore, we analysed the colour composition of cells infected with these three viruses at different multiplicities. We estimate that fewer than seven incoming genomes are expressed per cell. In addition, those templates that are expressed are the genomes selected for replication and packaging into virions. This finite limit on the number of viral genomes that can be expressed is an intrinsic property of the infected cell and may be influenced by viral and cellular factors. The Herpesviridae comprise a large family of DNA viruses that induce miscellaneous symptoms from unnoticed infection to a life-threatening disease in their hosts [1] . All herpesviruses have a unique virion structure and share a common replication strategy [2] . They replicate their DNA inside the host nucleus in distinct foci known as replication compartments [3] . To establish a replication compartment, nucleocapsids released into the cytoplasm after particle attachment and entry must move to the nucleus, and the viral genome must be released through nuclear pores. Depending on the efficiency of these processes, some fraction of infectious virions will establish a successful infection. This may be one of the causes for the high particle to plaque-forming unit (PFU) ratio of herpesviruses (ranging from 50 to 40,000 for different herpesviruses [1] , [4] ). Importantly, it is not clear after infection of a cell with many PFUs (a high multiplicity of infection, MOI), if all available genomes can be expressed or if there is a limit to the number of genomes that can be expressed and replicated. Pseudorabies virus (PRV) is a neuroinvasive swine alphaherpesvirus that infects most mammals, except for higher primates. Its propensity for controlled spread in the nervous system has led to its use in neural circuit tracing [5] , [6] , [7] , [8] , [9] , [10] . The less pathogenic PRV Bartha strains are favoured viral tracers, and derivatives have been constructed that express a variety of reporter genes facilitating visualization of infected cells [11] , [12] , [13] , [14] . Stochastic choice of expression among three or more different fluorescent proteins (FPs) enables labelling cells with many hues. Lichtman et al . used this idea to address neuronal connectivity. They developed a set of transgenic mice ('Brainbow mice'), in which each neuron expresses a different set of FPs allowing the differentiation of adjacent neurons by colour [15] , [16] . This method is based on DNA constructs (Brainbow cassettes) with open reading frames encoding three or four different FPs, and arranged in such a way that each FP is expressed by a random recombination event catalyzed by the Cre recombinase. We combined the multicolour properties of the Brainbow system with the tracing capabilities of PRV derivatives in a recombinant pseudorabies virus (PRV263) carrying a Brainbow cassette. Preliminary neuronal circuit tracing studies using PRV263 in Cre-expressing rats revealed a surprising number of single-coloured neurons that were in synaptic contact with Cre-expressing neurons (Card J.P., O.K. and L.W.E., unpublished results). This result suggested that only a small number of PRV genomes were spreading from Cre-expressing neurons to pre-synaptic neurons. Here, we use PRV263 and its derivatives to demonstrate that only those genomes that are expressed are packaged into progeny virions. Using this fact, we further demonstrate that an average of <7 incoming genomes are expressed per cell. Our finding may reflect an evolutionary mechanism to control viral population diversity. Construction of the Brainbow herpesvirus We constructed new PRV tracing viruses based on the multicolour approach of the Brainbow technology described by Lichtman et al . [16] for labelling neuronal circuitry in Cre-expressing transgenic mice [15] , [16] . We inserted the Brainbow 1.0L cassette into the gG gene in the PRV Bartha genome by homologous recombination producing the strain PRV263 (for details see Methods). When PRV263 infects a Cre-expressing cell, Cre-dependent recombination results in removal of the dTomato FP gene and the subsequent expression of either yellow (EYFP) or cyan (mCerulean) FPs, depending on recombination of different pairs of lox sites. Importantly, each viral genome can undergo only one Cre-dependent recombination event, thereby fixing the FP expressed by the recombinant. We tested the efficiency of recombination at either pair of lox sites during a single-step growth curve analysis of PRV263 on Cre-expressing PK15 cells (PK-Cre). Following infection of PK-Cre cells, progeny viruses were collected and assayed for their plaque-colour phenotype. As expected, Cre recombination resulted in three different progeny viruses, each expressing only one FP ( Fig. 1a ). Recombination occurs soon after infection and is efficient, with ∼ 44% of the progeny viruses expressing cyan and 36% expressing yellow FPs ( Fig. 1b ). 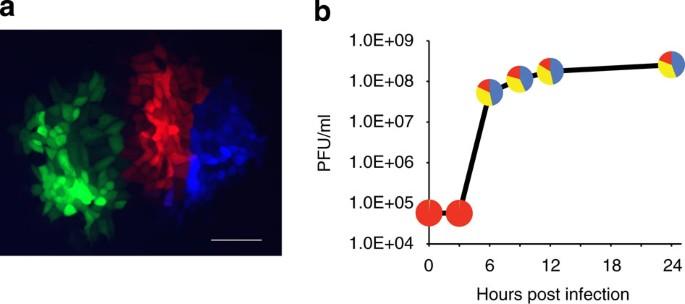Figure 1: Brainbow virus infection of PK-Cre cells. PK-Cre cells were infected with PRV263 at an MOI of 10, and at different time points post-infection, progeny viruses were collected and assayed for titre and colour. (a) Three adjacent plaques derived from progeny viruses express a single fluorescent protein: EYFP in green, dTomato in red and mCerulean in blue. Scale bar ,100 μm. (b) Each pie-chart point represents the ratio between red, cyan and yellow plaques at each time point. An average of three technical replicates is shown. In each replicate at least 250 plaques were counted. The differences between the replicates were very small. These results also confirm that each pair of Lox sites recombines with similar order of efficiency [17] (see also Table 1 , 34% yellow-only and 35% cyan-only plaques). Figure 1: Brainbow virus infection of PK-Cre cells. PK-Cre cells were infected with PRV263 at an MOI of 10, and at different time points post-infection, progeny viruses were collected and assayed for titre and colour. ( a ) Three adjacent plaques derived from progeny viruses express a single fluorescent protein: EYFP in green, dTomato in red and mCerulean in blue. Scale bar ,100 μm. ( b ) Each pie-chart point represents the ratio between red, cyan and yellow plaques at each time point. An average of three technical replicates is shown. In each replicate at least 250 plaques were counted. The differences between the replicates were very small. Full size image Table 1 Multiplicity dependence of cell colour within infectious centre plaques. Full size table Multicoloured segregation in PRV263 infectious centre plaques We used cultured non-neuronal porcine epithelial cell lines (PK15 cells) to explore this idea further. PK-Cre cells infected with PRV263 were plated on monolayers of non-Cre-expressing PK15 cells. Plaques arising from plating an infected cell onto an uninfected monolayer were termed 'infectious centre plaques' to contrast them from plaques derived from plating dilutions of virus stocks on uninfected monolayers. We observed that infectious centre plaques were multicoloured with distinct single-coloured sectors ( Fig. 2a ). This result was unexpected because localized cell-to-cell infection is thought to involve many virions. As many as 1,000 infectious PRV particles can be produced per cell [18] . If hundreds of viral particles emerge from the Cre-expressing cell and all their genomes are expressed in each of the adjacent cells, then all cells in such an infectious centre plaque will have similar fluorescent profiles: they should be infected by a similar average distribution of particles. In the other extreme, if only a single viral genome is transmitted and/or expressed in the adjacent cell, then the infectious centre plaque will comprise cells that express only one FP (pure colour cells). We observed neither plaque phenotype. 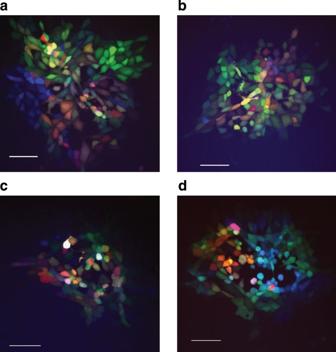Figure 2: Infectious centre plaques arising from Brainbow viruses. PK-Cre cells were infected with PRV263 (a,b) or PRV265 (c,d) at an MOI of 10 for 3 h. A small number of these infected cells were placed on monolayers of non-Cre PK15 cells. Two different infectious centre plaques (a,borc,d) arising from two different PK-Cre cells were visualized 24 h after plating. All images are coloured in RGB, and scale bars, 100 μm. Our results are more consistent with the hypothesis that each cell in the infectious centre plaque transmits and/or expresses a small number of viral genomes, because we observed that each cell has a unique fluorescent profile (non-pure colour), as seen in the infectious centre plaques shown in Figure 2a,b and in the Supplementary Movie 1 . A striking observation was that in many infectious centre plaques, one or more cells express a single pure colour, indicating that only a single type of genome is expressed. Figure 2: Infectious centre plaques arising from Brainbow viruses. PK-Cre cells were infected with PRV263 ( a , b ) or PRV265 ( c , d ) at an MOI of 10 for 3 h. A small number of these infected cells were placed on monolayers of non-Cre PK15 cells. Two different infectious centre plaques ( a , b or c , d ) arising from two different PK-Cre cells were visualized 24 h after plating. All images are coloured in RGB, and scale bars, 100 μm. Full size image Cre recombination is a very early event in infected cells When viral genomes enter cell nuclei, immediate early viral proteins are expressed, which in turn, facilitate expression of viral early proteins. Viral DNA replication can only occur in the presence of these early proteins. It is possible to determine whether Cre recombination occurs before or after DNA replication by examining the FP expression profile of the cells in an infectious centre plaque after low or high MOI. By limiting replication to one PFU per cell on average (low MOI) and if recombination occurs early before replication, most progeny virions will express a single FP. However, if recombination occurs later, during or after replication, many different recombinants will be packaged and the resulting progeny will be a mixture of yellow, cyan and red FP expressing virions. As indicated in Table 1 , we find that Cre recombination occurs early before significant replication is achieved. When PK-Cre cells are infected at low MOI, most cells in infectious centre plaques express the same single FP. Only 15% of these infectious centre cells are red, indicating that at least 85% of the cells have experienced one recombination event. When PK-Cre cells are infected with an average of several virions (high MOI), many more cells experienced at least one recombination event ( ∼ 93% overall). These results suggest that incoming genomes are active substrates for Cre recombination, but that after replication initiates, the viral genomes have low probability to recombine. Interestingly, under high MOI conditions more cells have viral genomes that did not recombine (>70% of the cells still express red with or without other FPs compared with <30% of red cells for low MOI infections). This observation probably reflects the saturation of Cre by the high number of incoming genomes. Wild-type PRV shows similar rapid colour segregation To determine whether this rapid segregation of FP expression during cell–cell spread is a property of the attenuated PRV Bartha strain background (PRV263), we inserted the Brainbow 1.0L cassette into the virulent PRV Becker genome producing PRV265 (see Methods for details). Infectious centre plaques originating from PRV265-infected PK-Cre cells show a similar sectoring phenomenon as seen for PRV263 infectious centre plaques (compare Fig. 2c,d with Fig. 2a,b ). We conclude that the rapid segregation of FP expression also occurs during wild-type PRV Becker infection and is not a unique property of the attenuated PRV Bartha background. Only a few viral genomes are expressed during infection The colour segregation phenomenon in infectious centre plaques may be transient and with time, all genomes in the infected cells may express all colours. Alternatively, colour segregation may be stable if only a few genomes are expressed during the entire infectious cycle. Supplementary Movies 1 and 2 of infectious centre plaques arising from a Cre-expressing cell reveal that each infected non-Cre-expressing cell maintains the same unique fluorescent profile throughout the entire process of plaque formation (although the intensity increases as infection proceeds). This result indicates that the ratio of expression of the different infecting viral genomes remains constant during the entire replication cycle. This phenomenon of constant expression level is an important finding, because it enables us to analyse fluorescent profiles of cells at a single point in time and to deduce the number of genomes contributing to the profile. Expressed genomes are replicated and packaged into virions The finding that coloured sectors within a plaque ( Fig. 2 ) do not change may indicate either that viral genomes contributing to the unique colour of an infected cell are the same genomes that replicate and give rise to progeny that infect neighbouring cells, or that the viral genomes establish spatially segregated, clonal replication compartments in the infected cell nucleus and progeny viruses egress directionally from these compartments to the surrounding cells. If the first possibility is true, the viral progeny of an infected cell will reflect the colour of the infected cells. To this end, we purified single-colour progeny viruses derived from PRV263 after exposure to Cre ( Fig. 1a ). These three isogenic strains differ only in the FP expressed. We then infected PK15 cells with equal numbers of virions that express either red or yellow FPs at either MOI of 10 or 100. Six hours post-infection (HPI), we sorted the infected cells according to their colour as detected by fluorescence-activated cell sorting (FACS) ( Fig. 3a,b ). These sorted cells were then incubated further and progeny virions were collected and plated for single plaques. We observed that with either lower or higher MOI infection, sorted red cells produced predominantly red progeny, sorted yellow cells produced mainly yellow progeny and sorted mixed coloured cells produced appropriate numbers of red or yellow progeny ( Fig. 3c,d ). Similar results were obtained from sorting of PRV263-infected Cre-expressing cells. We conclude that the limited numbers of genomes expressing their FPs also are those genomes being replicated and packaged. A similar idea was reported for HSV-1 infections, in which transcription and replication colocalize at early times after infection, while at later times, replication-only sites appear [19] . 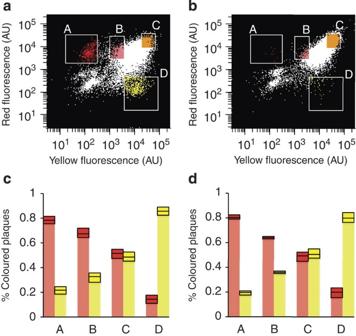Figure 3: Progeny viruses correlate with the colour of infected cell. PK15 cells were infected with equal amounts of red and yellow viruses originating from PRV263 at MOI of 10 (a,c) or 100 (b,d). Six HPI, the cells were sorted by FACS into four groups according to their colour spectra. Group A represent cells that highly express red fluorescence and low yellow fluorescence, group B represent cells that highly express red fluorescence and intermediate levels of yellow fluorescence, group C represent cells that highly express both red and yellow fluorescence and group D represent cells that highly express yellow fluorescence and low red fluorescence. (a,b) Results of one of three technical replicates are shown. Sorted cells were put back in culture and 24 h later, progeny were collected and plated for single plaques. Plaques were counted and colour determined using an epifluorescence microscope. (c,d) For each sorted population, the percentages of red and yellow plaques are represented by bars in the corresponding colour. The average of three different technical replicates and the range among the different replicates are presented by the outlined boxes. More than 150 plaques were counted for each sorted population in each replicate. Figure 3: Progeny viruses correlate with the colour of infected cell. PK15 cells were infected with equal amounts of red and yellow viruses originating from PRV263 at MOI of 10 ( a , c ) or 100 ( b , d ). Six HPI, the cells were sorted by FACS into four groups according to their colour spectra. Group A represent cells that highly express red fluorescence and low yellow fluorescence, group B represent cells that highly express red fluorescence and intermediate levels of yellow fluorescence, group C represent cells that highly express both red and yellow fluorescence and group D represent cells that highly express yellow fluorescence and low red fluorescence. ( a , b ) Results of one of three technical replicates are shown. Sorted cells were put back in culture and 24 h later, progeny were collected and plated for single plaques. Plaques were counted and colour determined using an epifluorescence microscope. ( c , d ) For each sorted population, the percentages of red and yellow plaques are represented by bars in the corresponding colour. The average of three different technical replicates and the range among the different replicates are presented by the outlined boxes. More than 150 plaques were counted for each sorted population in each replicate. Full size image The expression of only a small number of infecting genomes The rapid segregation of colours during cell–cell spread (plaque formation) may reflect either the passage of a small number of viral particles between cells or expression of FPs from only a few of the incoming genomes. We could distinguish between these possibilities by analysing the colour spectrum of single cells infected with three isogenic strains (PRV263 derivatives), each expressing a different FP. We used an equal mixture of three isogenic viruses expressing red, cyan or yellow FPs and infected cells at various MOIs ( Fig. 4 ). The colours of more than 6,000 infected cells (per infectious condition) were determined using an epifluorescence microscope equipped with six colour filters, as described in the Table 2 . The colours of each cell were plotted barymetrically according to their position on a triangle plot. Each vertex represents a different colour with single colour at each vertex, and two colour cells lie on the edges. As the MOI increases from low to high, cells should be infected with more genomes, and the colour of the infected cells should change from single colour to mixed colours. Unexpectedly, as MOI was increased, a significant number of cells were found on the edges of the colour triangle plots (representing single- and dual-coloured cells). Even with the highest MOI tested (MOI 100), the variability in colour spectrum among cells was large, even revealing a few single-colour cells (located at the triangle vertices). These data are striking because theoretically when 100 p.f.u. infect a cell, the probability of a single-colour infection is vanishingly small (probability of 3.3×10 −29 ). To be sure that these data were not particular for the attenuated PRV Bartha background, similar studies were carried out with the three different viral progeny arising after Cre recombination of the virulent strain PRV265 (each expressing a single FP). In these experiments, the variability in colour spectrum among cells was large, similar to the results obtained with PRV263 (compare Fig. 4a–e versus Fig. 4f–j ). 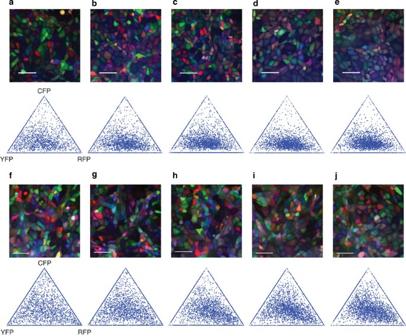Figure 4: High MOI infection with mixtures of three different single-colour viruses. We prepared stocks containing equal amounts of the parental virus and its two Cre recombinants for both PRV263 (a–e) and PRV265 (f–j). Both mixtures were used to infect a confluent plate of PK15 cells at different MOIs: 5 (a,f), 10 (b,g), 20 (c,h), 60 (d,i) and 100 (e,j). Six HPI, colour profiles of cells were visualized with an epifluorescence microscope. All images are coloured in RGB and scale bars, 100 μm. Each experimental condition (infections with one virus type and constant MOI) was replicated in three wells and the experiment was performed twice. The triangular plots represent the colour spectrum of more than 3,000 cells from three replicates (out of six; each cell is represented by a blue dot). Each vertex represents a different pure colour and points in between represent various mixtures of the colours. Therefore, cells expressing a single colour are found at the vertices, and cells expressing two colours are found on the edges. Cells with different mixtures of three colours are found inside the triangle. CFP, cyan FP. Figure 4: High MOI infection with mixtures of three different single-colour viruses. We prepared stocks containing equal amounts of the parental virus and its two Cre recombinants for both PRV263 ( a – e ) and PRV265 ( f – j ). Both mixtures were used to infect a confluent plate of PK15 cells at different MOIs: 5 ( a , f ), 10 ( b , g ), 20 ( c , h ), 60 ( d , i ) and 100 ( e , j ). Six HPI, colour profiles of cells were visualized with an epifluorescence microscope. All images are coloured in RGB and scale bars, 100 μm. Each experimental condition (infections with one virus type and constant MOI) was replicated in three wells and the experiment was performed twice. The triangular plots represent the colour spectrum of more than 3,000 cells from three replicates (out of six; each cell is represented by a blue dot). Each vertex represents a different pure colour and points in between represent various mixtures of the colours. Therefore, cells expressing a single colour are found at the vertices, and cells expressing two colours are found on the edges. Cells with different mixtures of three colours are found inside the triangle. CFP, cyan FP. Full size image Table 2 Filter sets used for image acquisition. Full size table We note that mCerulean is not as bright as the other two FPs [20] . As a result, cyan was difficult to distinguish from the background as seen in the triangle plots. This effect was more obvious in the Bartha-derived strains (PRV263), probably reflecting the fact that during Bartha infection, cells do not round up at 6 HPI (compared with the infection by virulent PRV265). As a result, the FPs were distributed over a larger area in PRV263-infected cells, which resulted in reduced overall fluorescence. To estimate the effect of this phenomenon on our analysis, we compared the number of single-colour cells in PRV263 and PRV265 infections. On average, there was a trend towards a lower number of cyan-only expressing cells (compare with other single-colour cells) at all MOIs in the PRV263 experiments only; however, this difference was not significant. Accordingly, we suggest that the brightness of the cyan FP has little effect on our ability to distinguish the cyan FP contribution to cell colour. Finally, we found that the colour segregation phenomenon was not specific to PK15 cells, as preliminary data indicate that similar colour profiles were obtained when primary embryonic rat neurons or primary embryonic mouse fibroblasts were infected. It seems likely that an intrinsic property of any infected cell type limits the number of genomes expressed. An estimation of the number of viral genomes being expressed We developed a model to estimate the number of PRV genomes expressed in each infected cell under different conditions (see Methods for details). Briefly, we define λ as the average number of genomes expressed in each cell. We assume that λ can be best represented as a Poisson random variable. Under each experimental condition (different MOIs, PRV263- or PRV265-derived viruses), we determined the number of distinct FPs (that is, zero, one, two or three) expressed in each infected cell. By counting >1,000 cells per well, we estimated λ by maximum-likelihood analysis, according to the following function: in which r 1 , r 2 and r 3 represent the numbers of one-colour, two-colour and three-colour cells, respectively, and n represents the total number of coloured cells. We then plot λ (average of six-well per condition) as function of MOI ( Fig. 5 ). 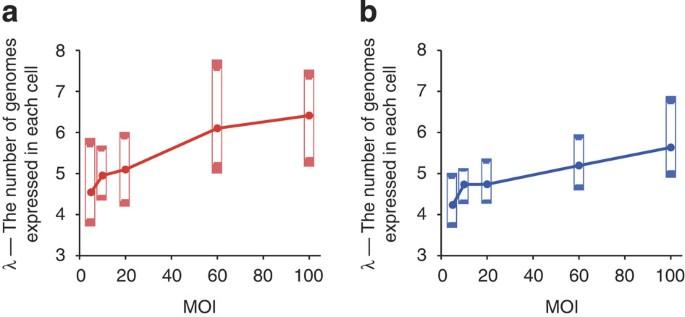Figure 5: A limited number of incoming genomes (λ) are expressed and replicated in a newly infected cell. Theλ-values for PRV263 derivatives (a, red) and for PRV265 derivatives (b, blue) are plotted as function of MOI. Each point represents theλ-value calculated from the average of two experiments (each experiment consists of data from three separate, replicate wells). The range of the calculatedλ-values among the different replicates is presented for each point by the outlined bar. Figure 5: A limited number of incoming genomes ( λ ) are expressed and replicated in a newly infected cell. The λ -values for PRV263 derivatives ( a , red) and for PRV265 derivatives ( b , blue) are plotted as function of MOI. Each point represents the λ -value calculated from the average of two experiments (each experiment consists of data from three separate, replicate wells). The range of the calculated λ -values among the different replicates is presented for each point by the outlined bar. Full size image Our analysis confirms that at high MOI, where hundreds of virions are available for uptake by the cell (see Methods section), fewer than seven PRV263 genomes and fewer than six PRV265 genomes are expressed on an average in each infected cell. The quantitative approach allows us to detect a similar increasing pattern of λ as function of MOI, for both viruses. These curves likely represent the combination of two separate limiting events. At lower MOI (<10), the predominant effect is the presence of sufficient viruses to establish infection in the cells. At high MOI (>10), a mechanism predominates that prevents expression of most entering genomes. We note that a constant λ -value for high MOI is not reached. This fact may reflect the limit of our experimental conditions (higher MOIs are difficult to achieve), or because there is a continuous decreasing effect of MOI on λ . It is interesting that a significantly higher number of the attenuated PRV263 derivative genomes are expressed compared with the more virulent PRV265 derivatives at high MOI: 6.1 compared with 5.2 for MOI 60, and 6.4 compared with 5.6 for MOI 100. As discussed above, the lower intensity of cyan FP may be one of the causes for this difference. We note that by 6 HPI at 100 MOI, PRV263 grows to higher titres when compared with PRV265 (3.5×10 7 compared with 1.5×10 6 , respectively), which is consistent with more PRV263 genomes being expressed. It may be that the more virulent PRV265 genome encodes viral gene products that regulate the number of genomes expressed and these functions are less active in the PRV263 background. PRV263 was designed to be a new viral tool for circuit tracing studies in neuroscience. The use of this Cre-conditional expression system allows a selective identification of subpopulation of neurons within neural circuits by their colours (Card J.P., O.K. and L.W.E., unpublished results). In our characterization of the expression of a Brainbow cassette by PRV, we identified an inhibitory process that limits expression and replication of incoming PRV genomes. Earlier work with PRV and herpes simplex virus-1 (HSV-1) had suggested that not all available genomes are replicated, but the mechanisms involved were not identified [21] , [22] . In addition, many viruses encode mechanisms to block superinfection by similar genomes (superinfection exclusion). One such mechanism is well known for the alpha herpes viruses. In this case, exclusion results after expression of gD, a viral glycoprotein essential for virion entry. In the infected cell, gD binds a cellular receptor and effectively renders the cellular receptor inactive, such that infection by other herpes virions is highly inefficient [23] , [24] , [25] , [26] , [27] . In addition, HSV-1 gD can induce internalization of receptors very early during infection [28] . Earlier studies with other alphaherpesviruses, including PRV, suggest that superinfection exclusion occurs by 4 to 6 HPI [13] , [29] . The phenomenon we observe cannot be classical superinfection exclusion, because it occurs early and, more importantly, is easily seen after high MOI infection of single cells, where no second rounds of infection (and therefore no superinfection) occur. The limitation of expression and replication of incoming viral genomes may reflect a bottleneck in one or more steps, including viral entry to the cell, nucleocapsids reaching the nucleus, release of viral genome into the nucleus or establishment of early replication centres 1. Although our study cannot identify the particular bottleneck, earlier work with HSV-1 suggests that many viral genomes can be observed in nuclei of infected cells (higher than the calculated MOI) and that not all of these genome complexes develop into replication compartments [30] , [31] , [32] . We therefore hypothesize that the bottleneck occurs after the genomes enter the nucleus. What happens to genomes that enter the nucleus but are not expressed and replicate? At the moment, we can only speculate as to their fate. Perhaps only the first genomes to enter the nucleus are the only ones that can establish replication compartments. It is clear that the unexpressed genomes cannot be activated by the replicating genomes in the same nucleus. These viral genomes could be degraded or could be silenced by cellular defense systems. Our findings correlate with the known association of viral genomes with proteins from the nuclear domain 10 bodies (ND10), which are limited in number in nuclei [33] , [34] . These complex structures, which contain many proteins, including PML, Daxx and Sp100, function as part of the intrinsic cellular defense system to block expression of foreign DNA [35] , [36] . Movement of some of the ND10 proteins towards herpesviral genome complexes results in a new ND10-like structure associated with the viral genome. Disruption of these new ND10-like structures is important for efficient viral replication [31] , [32] . The immediate early HSV-1 protein ICP0 (and its homologues in other alphaherpesviruses) has an essential role in inactivating ND10 structures and establishing viral replication compartments [37] , [38] . Using HSV-1 amplicons, Everett and colleagues [30] observed that genomes associated with ND10 proteins preferentially progress to form viral replication compartments and that each replication compartment initiates from one genome. Our data suggest that on average only 5–7 replication centres can be established, each originating from a single genome. Our model predicts that this number may vary for different cell types and can be modified by viral proteins, as we have observed for PRV263 and PRV265. In agreement with our results, Taylor et al . [39] found a small number of replication centres during HSV-1 infection of Vero cells. ND10 mediated, limited expression of invading viral genomes may be a general phenomenon for those viral genomes that replicate in the nucleus [34] . In addition, other cellular mechanisms may exist in other compartments to limit local expression of viral genomes. The simplicity of our method (three isogenic viruses each expressing a different FP) allows a similar test for the extent of genome expression for any viral genome that can stably express different fluorophores (including bacteriophages, RNA viruses and retroviruses). In summary, at low MOI (<5), infectious PRV particles entering cells have a relatively high probability for each genome ( ∼ 40% of the fluorescent-forming units (FFU)) to be expressed, replicated and packaged into virions. At higher MOIs (>10), most incoming viral genomes will not be expressed or replicated. The surprising limit of 5–7 genomes for expression and replication, independent of the number of infectious genomes entering the cell, suggests that viral gene products have evolved to regulate this process. Given that both productive and quiescent infections are the hallmark of all herpesviruses, such limiting expression may be an ancient acquisition in their evolution. In addition, perhaps this phenomenon represents a positive selection mechanism to enable sampling of all available genomes at early stages of host infection when few genomes are available. In contrast, during a successful infection (conditions of high MOI), limiting genome accessibility may maintain successful genomes by regulating diversity. Cell lines and virus strains The porcine kidney epithelial cell line PK15 was used to propagate and titre all viral strains. The PK-Cre was described previously [11] . The pBrainbow1.0L cassette was described previously [15] . This cassette encodes three different FPs, and depending on the Cre-recombinase activity only one of the three proteins can be expressed from the strong cytomegalovirus promoter. The unrecombined cassette expresses dTomato (red fluorescence), and no other colour. After Cre-mediated recombination at either of two pairs of lox sites, the red reporter DNA is excised and, depending on if loxP by loxP or lox2272 by lox2272 recombination occurs, a cyan (mCerulean) or yellow (EYFP) reporter will be expressed from the cytomegalovirus promoter. To construct PRV263 or PRV265, pBrainbow1.0L was linearized and co-transfected into PK15 cells with DNA from either PRV152, an attenuated PRV Bartha derivative expressing enhanced green fluorescent protein (EGFP), or PRV151 a wild-type PRV Becker derivative expressing EGFP [12] , [40] . The original EGFP cassette at the gG locus was replaced with the Brainbow cassette by homologous recombination. Resulting recombinants were plaque purified on PK15 cells by selection of red plaques. Measuring viral infectious units The number of PFUs per cell (MOI) was determined by counting the number of PFU in virus stocks on monolayers of PK15 cells. Each viral stock was titred at least four times and average titre was taken. Although the PFU is the most common measurement for viral titre, this measurement underestimates the actual number of viral genomes. We used two other methods to estimate the number of genomes infecting cells. First, as the Brainbow viruses expressed a single FP, we determined the number of FFUs in our stocks. We found that the FFU/PFU ratio is about 2.5 (for both PRV263 and PRV265). By this method, at an MOI of 100 p.f.u. per cell, ∼ 250 genomes are capable of expressing FPs. We next determined the number of DNA genomes/PFU in our stocks using reverse transcription–PCR with primers from the UL54 region for transcriptional analysis [41] (forward primer, 5′-TGCAGCTACACCCTCGTCC and reverse primer, 5′-TCAAAACAGGTGGTTGCAGTAAA). Our measurements suggest that the genome/PFU ratio is ∼ 10 to 20 (both for PRV263 and PRV265). By this method, at an MOI of 100 p.f.u. per cell, ∼ 1,000 to 2,000 genomes enter cells. Taken together, these findings confirm that there are more viral genomes than PFUs. Importantly, the genome/PFU ratio should be constant, but the bottleneck in expression of incoming genomes we observed is nonlinear; the percent of expressing genomes decreases as MOI increases. Cell sorting PK15 cells were infected either at an MOI of 10 or 100 with equal amounts of red and yellow viruses originating from PRV263. Six hours later, cells were washed with citrate buffer at pH 3 to inactivate any free viruses. Cells were then trypsinized from the dish and kept on ice until sorted. A total of 200 cells were sorted for each group using FACSVantage SE w/DiVa (BD Biosciences) cell sorter. The sorted cells were incubated for 24 h at 37 °C to complete the replication cycle. Resulting infectious virions released in the medium were collected and plated on PK15 cells for single plaques and colour determination. Microscopy All images and movies were taken using a Nikon Eclipse Ti-E epifluorescence inverted microscope. Image acquisition To estimate the number of PRV genomes expressed in each infected cell, we first obtained images of cells infected with equal amounts of three viruses (each expressing a different FP) using Nikon Eclipse Ti-E epifluorescence inverted microscope. We carried out infections with two PRV backgrounds with identical Brainbow cassettes (PRV263, PRV265) and five different MOI (5, 10, 20, 60 and 100). Each experimental condition (infections with one virus type and constant MOI) was replicated in three wells and the experiment was performed twice. From an individual well, five random areas were imaged. The images were taken using six different filter sets (Chroma Technology) as detailed in Table 2 . To calibrate our system, we determined the spectrum profile of cells infected at an MOI of 20 with virus expressing single FP. Two wells for each virus were imaged (one in each experiment). Image processing To determine the number of colours (1, 2 or 3) in each infected cell, we processed the infected cell images in four steps. First, we manually marked the centres of the cells using the NIS Elements software (NIKON Instruments). We marked at least 200 cells from every image (average of 237.5 cells per image). The fluorescence intensity from all six filters, as well as the coordinates of the each cell centre, was collected. Similarly, we marked at least 10 background areas in each image. Second, to reduce low-frequency noise due to experimental conditions, we used the 10 background intensity levels for predicting overall background values, varying smoothly spatially over the image. This calculation was done with Thin-Plate-Splines two-dimensional interpolation. Then, we subtracted the predicted background values from all cellular intensity measurements in the image. Third, we estimated the red (for dTomato expression), green (for EYFP expression), and blue (for mCerulean expression) colour intensities for each cell using the data from each of the six filters. We then used the single-colour virus spectrum profile for each pure colour infection to decompose, by a least squares fitting procedure, each of the six fluorescence intensities to RGB magnitudes. Fourth, we determined the number of expressed colours in each infected cell. This was performed, for every cell, by counting how many colours (zero, one, two or three) were above a threshold value. We used different thresholds for each colour channel, which were determined by analysing the single-colour virus infections. For example, to set the red threshold, we analysed the cells' red values obtained from both the single-blue and single-green viral infections and took 2 s.d.s above the mean of this distribution. Mathematical model We have constructed a mathematical model for estimating the number of incoming viral genomes, given the distribution of cell colours across the experiments. Intuitively, the larger the number of expressing viral genomes, the smaller the number of single-coloured and double-coloured infected cells should be observed. Cells were infected for six hours at high MOI (>5) allowing synchronized infection. Under these conditions, secondary infection from new progeny viruses is effectively precluded. We did not observe any evidence of exclusion after high MOI infection. Therefore, we conclude that each virus can independently infect a cell. Given these facts, we assume that the number of incoming viral genomes can be represented as Poisson random variable. Let X ∼ Poisson( λ ) denote a random variable counting the number of incoming viral genomes expressed in a single cell. We wish to estimate λ , the average number of incoming viral genomes being expressed, based on our experiments. Although we cannot directly sample the random variable X , we can sample a related random variable Y defined as the number of colours (that is, zero, one, two or three) expressed in an infected cell. The key observation of this paper is that with enough samples of Y from different cells, one can determine X . Therefore, we can estimate λ in a robust way. First, we compute the different probabilities of Y . We start with zero colour cells For single colours we have In a similar way, Combining all the above, we get the formula In our setting, we assumed that the random variables Y i , i =1,2,..., n , reflecting the number of colours in the infected cells, are independent. To estimate the model parameter λ , we performed maximum-likelihood analysis. Denote by r 0 , r 1 , r 2 , r 3 the number of zero-coloured cells, single-colour cells, double-colour cells and triple-colour cells, respectively (measured from the data as explained in previous sections); we have r 0 + r 1 + r 2 + r 3 = n . Further, denote by r ( i ), i =1, 2, ..., n , r ( i )=0, 1, 2 or 3, the observed number of colours, in the experiments, for the individual cells. The log-likelihood function is This equation is used to extract the parameter λ as follows: (1) we count the number of none, single-, double- and triple-colour cells, and (2) substitute into the equation and determine the maximizing λ ; this maximizing λ is given by the following equation: This λ is the most likely one under our assumptions. How to cite this article: Kobiler, O. et al . Herpesviruses carrying a Brainbow cassette reveal replication and expression of limited numbers of incoming genomes. Nat. Commun. 1:146 doi: 10.1038/ncomms1145 (2010).